Ballistic interferences in suspended graphene The low-energy electronic excitations in graphene are described by massless Dirac fermions that have a linear dispersion relation. Taking advantage of this ‘optics-like’ electron dynamics, generic optical elements like lenses and wave guides have been proposed for electrons in graphene. Tuning of these elements relies on the ability to adjust the carrier concentration in defined areas. However, the combination of ballistic transport and complex gating remains challenging. Here we report on the fabrication and characterization of suspended graphene p – n junctions. By local gating, resonant cavities can be defined, leading to complex Fabry–Pérot interferences. The observed conductance oscillations account for quantum interference of electrons propagating ballistically over distances exceeding 1 μm. Visibility of the interferences is demonstrated to be enhanced by Klein collimation at the p – n interface. This finding paves the way to more complex gate-controlled ballistic graphene devices and brings electron optics in graphene closer to reality. The wave nature of any physical entity, be it light or electrons, is demonstrated by measuring an interference pattern in an apparatus called interferometer. We distinguish two types of interferometers: two-path and multi-pass interferometers. Examples for the former are the Michelson and the Mach–Zehnder interferometer, which are both widely used in optical experiments. In contrast, the Fabry–Pérot (FP) interferometer is of the multi-pass type. In optics, an FP interferometer is an element that consists of a transparent glass plate with two partially reflective surfaces on opposite sides. It can therefore be viewed as a cavity. Light within the cavity is bouncing back and forth between the mirrors, but at each reflection a fraction of light is coupled out. The superposition of all outgoing waves gives rise to an intensity modulation (the interference pattern) that depends on the wavelength of the light and the distance between the mirrors. In solid-state physics, a two-dimensional (2D) conducting sheet between two electrodes could realize an electronic FP interferometer. However, the mean free path (mfp) and phase-coherence length are usually much shorter than the device size leading to purely diffusive incoherent electronic transport. Before the advent of one-dimensional (1D) and 2D carbon allotropes, long mfps and optics-like experiments have only been realized in complex semiconductor heterostructures [1] , [2] . During the last decade, the long mfp (several hundreds of nanometres) accessible in low-dimensional carbon materials enabled one to explore different ballistic phenomena. In particular, FP interferences have been demonstrated in carbon nanotubes [3] and graphene nanostructures [4] , [5] , [6] . In the former case, interferences were observed over a distance as long as 0.5 μm, whereas the cavity size was <100 nm in the latter. Nowadays, graphene junctions show a mfp close to 1 μm [7] , and electron guiding [8] as well as transverse magnetic focusing have been revealed [9] . However, even if graphene appears as a perfect platform for electron optics [10] , [11] , [12] , [13] , quantum interferences with long mfp >1 μm and complex electrostatic gating still remain to be demonstrated. In this article, we report FP interferences in a gate-tunable monolayer graphene p–n junction 1 μm long with coherent ballistic electron motion. We observe an interference pattern in both the unipolar and bipolar regime and for all combinations of cavity mirrors, either defined at the source and drain contacts or at a p–n junction in the middle of the device. Ideal graphene FP cavity In graphene, charge carriers with small quasi-momentum ħ k counted from the corner of the Brillouin zone have a linear dispersion [14] , [15] , [16] . In the conduction and valence band, the energy E ( k ) as a function of wavevector k is given by E c ( k )= ħν F k and E v ( k )=− ħν F k , respectively, where k =| k | and ν F is the Fermi velocity; see Fig. 1a . Electron number density n is given by n =sgn( E ) k 2 / π . Taking a ballistic graphene cavity, as sketched in Fig. 1b , the phase difference between two successive outgoing rays is Δ φ =2 kL cos( θ ), where L is the size of the cavity and θ the angle of incidence of the electron waves relative to the normal of the mirror. 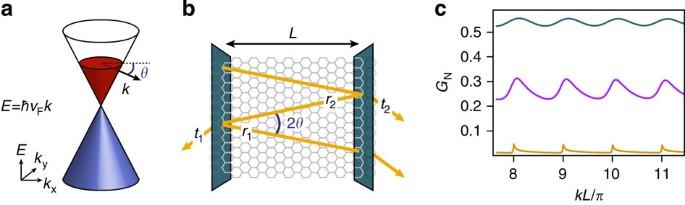Figure 1: Ideal graphene FP cavity. (a) Low-energy dispersion in pristine graphene. (b) Sketch of an idealized graphene FP resonator. (c) Normalized conductance through an ideal graphene cavity as a function of the dimensionless parameterkFL/πfor three different finesses:F=1,600 in yellow,F=4.9 in purple andF=0.4 in blue. Summing over all partial outgoing waves, one obtains for the transmission probability [17] : Figure 1: Ideal graphene FP cavity. ( a ) Low-energy dispersion in pristine graphene. ( b ) Sketch of an idealized graphene FP resonator. ( c ) Normalized conductance through an ideal graphene cavity as a function of the dimensionless parameter k F L / π for three different finesses: F =1,600 in yellow, F =4.9 in purple and F =0.4 in blue. Full size image where F =4| r 1 || r 2 |/| t 1 | 2 | t 2 | 2 , with | r 1,2 | and | t 1,2 | as the reflection and transmission amplitudes at the two interfaces, respectively. F is a measure of the quality factor and known as the finesse. The finesse of an FP interferometer determines the visibility of the interference pattern, that is, the difference in T between constructive and destructive interference relative to the mean transmission probability. The visibility is very close to unity if , and it is small and given by F in the opposite limit. As the electric measurement of the graphene conductance cannot distinguish the direction of the waves within the cavity, one has to integrate over the angles to deduce the expected visibility for the conductance ( G max – G min )/( G max + G min ). The normalized dimensionless conductance is shown in Fig. 1c as a function of the dimensionless parameter kL/π for three cases ( r 1 = r 2 =0.8, F =1,600), ( r 1 = r 2 =0.4, F =4.9) and ( r 1 = r 2 =0.2, F =0.4). For all three cases, resonances appear equidistantly whenever k F L is a multiple of π , indicating that the conductance peaks are mainly because of electrons at small incident angles (see Supplementary Fig. S1 and Supplementary Note 1 ). We now focus on a graphene FP cavity that consists of two segments: left and right. We assume that in both segments the carrier density and its sign ( n and p ) can be controlled independently by two-gate voltages V left and V right with identical efficiency. 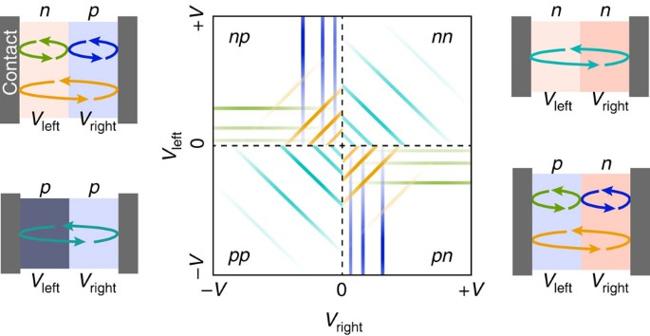Figure 2: Two ideal graphene FP cavities in series. Schematic representation of all possible resonance conditions (central panel) in a FP resonator that consists of two segments of equal size (left and right panels). The carrier density and carrier type (norp) in both segments can be tuned independently byVleftandVright. FP resonances may occur because of reflection at the outer contacts or at an internaln–p(p–n) interface between the two segments. The possible resonant conditions are indicated by colour-coded lines for the respective cases in the middle part. Figure 2 shows in a schematic 2D conductance map the expected FP interference patterns as a function of V left and V right . This map has four quadrants corresponding to the four polarity configurations [18] . If the left and right segments have the same polarity ( nn or pp ), the cavity is in the unipolar regime. In contrast, in the case of opposite polarities ( np or pn ), the cavity is in the bipolar regime. In the unipolar regime, only interferences of electrons bouncing back and forth between the two outer contacts are expected (lower left and upper right panel in Fig. 2 ). The corresponding beating pattern evolves along V left = V right and is indicated by the light-blue lines in the central panel of Fig. 2 . In the bipolar case, assuming a semi-transparent p–n interface between the segments, the junction can be considered as two cavities in series, each controlled by its respective gate. Resonances in the left (right) cavity depend only on V left ( V right ) and are represented by green (blue) lines. Another distinct set of resonances in the bipolar regime can arise from charge carriers that tunnel through the central p–n interface in the middle and bounce back and forth between the outer contacts. The corresponding beating pattern should evolve along the condition k left ≈ k right . In terms of gate voltages, this condition corresponds to V left ≈ − V right as indicated in Fig. 2 by the orange lines. Figure 2: Two ideal graphene FP cavities in series. Schematic representation of all possible resonance conditions (central panel) in a FP resonator that consists of two segments of equal size (left and right panels). The carrier density and carrier type ( n or p ) in both segments can be tuned independently by V left and V right . FP resonances may occur because of reflection at the outer contacts or at an internal n–p ( p–n ) interface between the two segments. The possible resonant conditions are indicated by colour-coded lines for the respective cases in the middle part. Full size image Device preparation To realize experimentally such a tunable FP cavity, devices were prepared by combining a mechanical transfer process [19] with a hydrofluoric acid-free suspension method proposed by Tombros et al . [20] The fabrication process is schematically shown in Fig. 3a . For a complete description, see Methods. Clean graphene was obtained by an in situ current annealing process. 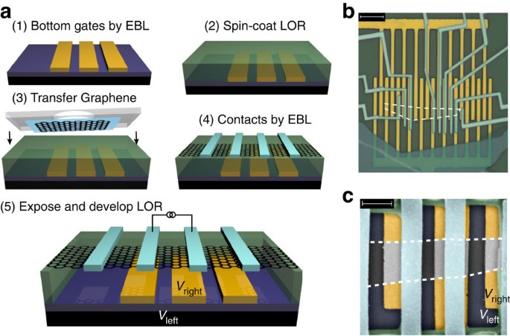Figure 3: Suspended graphene devices. (a) 3-dimensional illustration of the device fabrication consisting of the following steps: (1) bottom gates are realized by standard e-beam lithography on a doped Si wafer with 300-nm-thick SiO2top layer and (2) covered by a 700-nm-thick LOR (lift-off resist) layer. (3) Graphene is exfoliated on a separated wafer covered by a stack of polyvinyl alcohol/PMMA, and then aligned to the bottom gates and transferred. (4) Contacts to the graphene are then realized with standard e-beam lithography followed by an evaporation of 50 nm palladium. (5) Finally, the device is suspended by selectively exposing the LOR with a large dose and developing it. (b) Optical image of several junctions defined within the same graphene flake indicated by white dashed lines. Bottom gates are in yellow and ohmic contacts in blue. The LOR resist appears in dark green. Scale bar, 5 μm. (c) Scanning electron microscopic image of three graphenep–njunctions in a row. Bottom gates are shown in yellow and contacts in light blue. Scale bar, 1.2 μm. Figure 3b shows a coloured optical image of several junctions realized within the same graphene flake indicated by white dashed lines. A scanning electron microscopic micrograph of three p–n junctions is presented in Fig. 3c . A voltage applied on the bottom gate ( V right , yellow electrodes in Fig. 3b,c ) will tune the charge carrier density on the right side of a junction, whereas a voltage applied on the back gate ( V left ) will act on the left side. The device was measured in a 4 He cryostat at a temperature of T =1.5 K. Differential conductance, G = dI / dV was measured by standard lock-in techniques with a voltage bias of 100 μV at 77 Hz. Series and contact resistances were not subtracted from the data. Figure 3: Suspended graphene devices. ( a ) 3-dimensional illustration of the device fabrication consisting of the following steps: (1) bottom gates are realized by standard e-beam lithography on a doped Si wafer with 300-nm-thick SiO 2 top layer and (2) covered by a 700-nm-thick LOR (lift-off resist) layer. (3) Graphene is exfoliated on a separated wafer covered by a stack of polyvinyl alcohol/PMMA, and then aligned to the bottom gates and transferred. (4) Contacts to the graphene are then realized with standard e-beam lithography followed by an evaporation of 50 nm palladium. (5) Finally, the device is suspended by selectively exposing the LOR with a large dose and developing it. ( b ) Optical image of several junctions defined within the same graphene flake indicated by white dashed lines. Bottom gates are in yellow and ohmic contacts in blue. The LOR resist appears in dark green. Scale bar, 5 μm. ( c ) Scanning electron microscopic image of three graphene p–n junctions in a row. Bottom gates are shown in yellow and contacts in light blue. Scale bar, 1.2 μm. 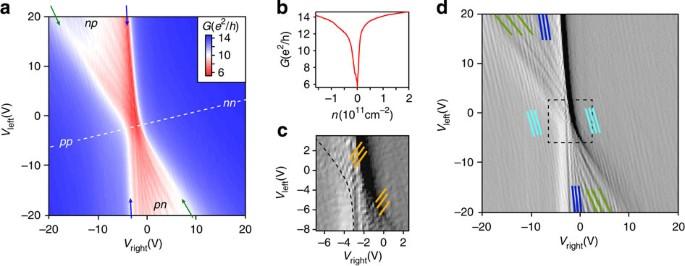Figure 4: Conductance of a suspendedp–ngraphene device. (a) Two-terminal differential conductanceG=dI/dVas a function ofVrightandVleftatT=1.5 K, demonstrating independent control of carrier type and density in the left and the right side of the graphene sheet. Labels in each of the four conduction regimes indicate the carrier type. (b) Conductance as a function of charge carrier densitynalong the dashed white line ofa. (c) Zoom into the transconductance map presented, ind, around the charge neutrality point. (d) Transconductance obtained from the numerical derivative with respect toVrightofaemphasizing conductance oscillations. Colour-coded lines link the observed conductance oscillations with the FP interference pattern expected from the simple picture ofFig. 2: light-blue lines in the unipolar regime, green and blue lines for interferences on either side of the graphene in the bipolar case and orange lines for full-length interference in the bipolar regime. Full size image Electronic transport characteristic Figure 4 shows the main experimental result of this work. In part (a), the differential conductance between the two contacts as a function of V right and V left is presented for a junction of length L =1.2 μm and width W =3.2 μm. As expected, this 2D plot reveals four regions indicated by the labels pp , nn , np and pn corresponding to different carrier types in the two sides of the sample. The borders between the unipolar and bipolar regions coincide with the charge neutrality point of the left and right graphene segments (indicated by blue and green arrows, respectively). The border lines between the different regions are not perpendicular to each other, as expected for independent gates and discussed above in Fig. 2 for two reasons. First, both the back gate and the bottom gate are at a distance to the graphene sheet that is comparable to the length of the device. This leads to a cross coupling between the two gates, that is, the right gate also affects the left graphene segment and vice versa . Second, the back gate (left gate) is below the bottom gates, and therefore is strongly screened by these, leading to a much weaker gate coupling from the back gate to the graphene than that from the bottom gate. Figure 4: Conductance of a suspended p – n graphene device. ( a ) Two-terminal differential conductance G = dI / dV as a function of V right and V left at T= 1.5 K, demonstrating independent control of carrier type and density in the left and the right side of the graphene sheet. Labels in each of the four conduction regimes indicate the carrier type. ( b ) Conductance as a function of charge carrier density n along the dashed white line of a . ( c ) Zoom into the transconductance map presented, in d , around the charge neutrality point. ( d ) Transconductance obtained from the numerical derivative with respect to V right of a emphasizing conductance oscillations. Colour-coded lines link the observed conductance oscillations with the FP interference pattern expected from the simple picture of Fig. 2 : light-blue lines in the unipolar regime, green and blue lines for interferences on either side of the graphene in the bipolar case and orange lines for full-length interference in the bipolar regime. Full size image A slice through the 2D conductance plot along the white dashed line is shown in Fig. 4b as a function of carrier density n , which we estimated from a parallel plate capacitor model. A positive sign refers to the n -region and a negative sign likewise to the p -region. A change in gate voltage of 1 V along the white dashed line induces a change in density of n ≈9 × 10 9 cm −2 . The graph exhibits a remarkably sharp conductance dip, corresponding to the charge neutrality in the entire graphene sheet. The fact that this dip also occurs close to zero gate voltage reflects the high quality of the graphene sample. The conductance saturation and the asymmetry at high carrier density suggest an n -type doping of the graphene contacts below the palladium contacts [21] , [22] . By defining the mobility as μ =1/ e × dσ / dn with σ the graphene conductivity, we estimated a mobility of μ ≈150 × 10 3 cm 2 V −1 s −1 at n =4 × 10 9 cm −2 . The junction reaches a minimal conductivity of σ min = G L / W ≈2 e 2 / h close to the ballistic limit of 4 e 2 / πh (ref. 23 ), indicating a weakly disordered graphene sheet [7] , [24] . Signatures of quantum interferences The most striking features in the conductance map are, however, the oscillation patterns visible in both the unipolar and bipolar configuration. To emphasize these features, the transconductance dG/dV right numerically calculated from the data in Fig. 4a is presented in Fig. 4d . The different interference patterns expected from the simple picture of Fig. 2 are well revealed in this map. In the unipolar case, one global interference pattern is visible (highlighted in a small region by light-blue lines) corresponding to FP interferences of electron waves that bounce back and forth between the outer metallic contacts. In the data, the density separation Δ n ≈10 10 cm −2 between constructive interference peaks at around n ≈10 11 cm −2 . On the basis of the equation n =sgn( E ) k 2 / π and the resonance condition Δ kL cavity = π , we derive the relation . This yields an effective cavity length L cavity ≈1.1 μm in good agreement with the geometrical length L =1.2 μm of the junction . In the bipolar regime at high doping, two clear oscillation patterns are visible. One pattern is mainly tuned by V right , indicating that resonances arise from the cavity created at the right side of the p–n interface. This pattern is highlighted by blue lines in Fig. 4d . The other pattern marked by green lines is predominantly tuned by V left , indicating that it originates from the cavity formed at the left side of the p–n interface. When applying a magnetic field perpendicular to the graphene flake, the electron trajectories are bent. Interference conditions are then modified such that the interference patterns disperse with the magnetic field. This effect has been previously studied in ref. 5 and is shown in both regimes (unipolar and bipolar) in Supplementary Fig. S2 and Supplementary Note 2 . The area in the transconductance map marked by the dotted square in Fig. 4d is enlarged in Fig. 4c . It shows yet another oscillation pattern (orange lines). It follows gates values such that n left ≈− n right with an interference period Δ n ≈3 × 10 9 cm −2 at n =10 10 cm −2 leading to L cavity ≈1.2 μm. We conclude that these oscillations must arise from quantum interference over the full device length, that is, charge carriers that tunnel through the p–n interface, changing their character from n to p and back. We emphasize at this point that there is no evidence of disorder in the transconductance plot of Fig. 4d . All patterns are regular and can be ascribed to distinct FP cavities, some of which extend in length over the whole device. The occurrence of FP interference patterns implies that the phase-coherence length exceeds at least twice the system size. Random disorder would then generate further interference patterns, but these are never regular. The fact that we can deduce from the interference pattern effective cavity lengths from contact to contact and that we do not see any irregular features are strong signs for ballistic coherent transport over distances exceeding 2 μm. Simulation and comparison with experiment To confirm the ballistic origin of the observed interference patterns, the charge transport through the graphene device is simulated in the phase-coherent ballistic regime using the actual geometrical parameters of the device (see Supplementary Figs S3 and S4 and Supplementary Note 3 ). The computed conductance is shown in Fig. 5d , which presents a purely ballistic tight-binding transport simulation using a real-space Green’s function method within the Landauer–Büttiker formulation [25] , combined with the quantum capacitance model for carrier density computation [26] . As no dephasing or energy averaging has been incorporated, the obtained conductance modulations show the maximal possible visibility for this device geometry. The correspondence between theory and experiment is remarkably good and supports the picture of ballistic motion drawn from experiment. However, a relatively clear discrepancy can be seen at low carrier density. The minimum conductance from the theory approaches zero, whereas it remains finite in the experiment. In the long wavelength limit (low carrier density), scattering at the edges of the graphene flake becomes relevant. As the suspended graphene is simulated by an ideal honeycomb lattice extending infinitely along the lateral dimension without any disorder, the present theory provides only the bulk component of the ballistic conductance and does not account for any edge effects on the transport. Thus, we conclude the discrepancy of the minimal conductance between experiment and theory to be attributed to the absence of the edges in the simulation. Nevertheless, our main focus is the bulk property of the suspended graphene that gives rise to the FP interference, and this discrepancy therefore does not influence our discussion. 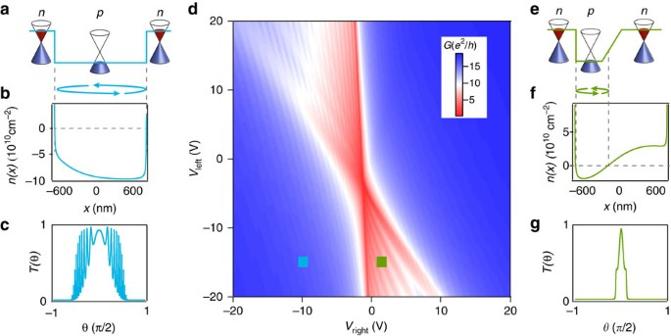Figure 5: Simulation of the suspended graphene device. (a) Schematic view of charge carrier configuration at the unipolar point (Vleft,Vright)=(−15,−10) V is indicated by a blue square ind. (b) Calculated charge carrier profile at this point and (c) associated simulated transmission function versus incident angleθ. (d) Conductance map obtained by tight-binding transport calculation as a function ofVleftandVright. (e–g) Same asa–cbut for parameters at the bipolar point (Vleft,Vright)=(−15,2) V is indicated by a green square ind. Figure 5: Simulation of the suspended graphene device. ( a ) Schematic view of charge carrier configuration at the unipolar point ( V left , V right )=(−15,−10) V is indicated by a blue square in d . ( b ) Calculated charge carrier profile at this point and ( c ) associated simulated transmission function versus incident angle θ . ( d ) Conductance map obtained by tight-binding transport calculation as a function of V left and V right . ( e – g ) Same as a – c but for parameters at the bipolar point ( V left , V right )=(−15,2) V is indicated by a green square in d . Full size image As pointed out before, we do see all the expected FP resonance patterns because of the formation of distinct cavities having different doping and different types of mirrors. However, the strength of the oscillation pattern (the visibility) varies in different regions. This is linked to the reflection properties of our cavity ‘mirrors’, determining the cavity finesse. Cavities can be created either by sharp or smooth unipolar or bipolar potential steps. Let us first consider a unipolar potential step. If d is the length over which the carrier density varies and k F the mean Fermi wavevector, the junction is assumed smooth if and sharp in the opposite limit. In the smooth case, the electrons follow adiabatically the potential evolution. They may bend similar to light rays in a medium with a slowly varying refractive index, but they will not backscatter. In contrast, for a sharp potential step one might expect backscattering. However, charge carriers in graphene are chiral, that is, they have a pseudospin that is intimately tied to the wavevector. Scattering from a state with wavevector k into − k is forbidden because this would flip the pseudospin. The conservation of pseudospin is only lifted, if the potential step is abrupt on the atomic scale [27] , which is not the case here. Thus, pseudospin conservation implies that effectively all unipolar potential steps are highly transmissive for almost every incident angle [28] (only electrons with incident angles close to π /2 have an appreciable backscattering probability). Cavities created by unipolar interfaces have consequently a small finesse and will display small visibilities. We turn now to the reflection properties of a p–n junction. We assume that the carrier densities on both sides are of opposite sign but equal in magnitude, and that k F denotes the wavevector in the homogeneous region outside the junction. In the case of a sharp p–n interface with , the transmission probability is given by T ( θ )=cos 2 ( θ ) (ref. 27 ). The corresponding cavities have a small finesse for electron waves over a large range of incident angles around θ =0, and will therefore have a small visibility. The situation is different for a smooth p–n junction. As the charge carrier density evolves smoothly through zero, essentially all electron trajectories are adiabatically refracted off the interface (total reflection) except for the normal one, which can Klein-tunnel through the junction [27] , [29] . The transmission probability through such a smooth p–n junction is given by the expression T ( θ )=exp(− πk F d sin 2 θ ) (ref. 27 ), which also predicts perfect transmission at normal incidence. Similar to the sharp interface, one could expect the visibility of the interference pattern to be small. However, Klein tunnelling does not only yield full transmission at normal incidence but also leads to a strong collimation in transmission. Therefore, almost all trajectories that are incident at a small angle ( θ ≠0) are exponentially suppressed and do not add to the total conductance. This suppression of the background current increases the overall visibility. Although the finesse vanishes for θ =0, the contribution from small angles (with θ ≠0) yields a higher visibility than the case for unipolar or sharp bipolar cavities (see Supplementary Fig. S5 and Supplementary Note 4 ). Visibility of the interference Based on the preceding discussion, we now compare the observed visibilities for two particular cases in (a) the unipolar and (b) bipolar regime at gate voltages ( V left , V right )=(−15,−10) V and (−15, 2) V, respectively. These two points are marked in Fig. 5d by light-blue and green squares. For both cases, the reflection properties at the contacts are important parameters and need to be known. The full comparison of the simulation with the experiment reveals that the contacts dope graphene as n -type. In addition to this doping, the simulation includes a small mass term in the contacted region [30] . For the unipolar case, the simulation yields the charge carrier density profile plotted in Fig. 5b . In this configuration, the interior of the FP cavity is p -type with mirrors created by the p–n interfaces close to the Pd contacts. The latter can be considered to be relatively sharp owing to the rapid decay of the contact-induced screening potential [31] (see Supplementary Figs S4 and S6 and Supplementary Note 5 ). Consequently, these interfaces are almost transparent and give rise to low finesse for the FP interferences as found in the experimental and the numerical conductance map with respective average visibilities of 0.5% and 2%. In the bipolar case, the simulation yields the carrier density profile plotted in Fig. 5f . It presents an extremely smooth p–n interface created electrostatically in the middle of the graphene sheet. The two cavities created on the right and left side will present a much higher finesse than in the unipolar configuration, which consistently leads to higher visibilities in both the experimental and numerical conductance maps. The average visibility for the experiment is around 5%, whereas the simulation yields 20%. The calculated angle-dependent transmission probabilities for both regimes are plotted in Fig. 5c,g , respectively, which clearly demonstrate that the visibility difference between the unipolar and bipolar regime is a direct consequence of the exponential collimation of Klein tunnelling [27] , [28] , [29] . In conclusion, we have fabricated and characterized a suspended graphene p–n junction. FP-type conductance oscillation patterns visible in both unipolar and bipolar regimes point to an extremely long mfp and phase-coherence length >2 μm accessible in our device. Good agreement of the tight-binding transport simulation with the experiment confirms the ballistic origin of the measured interference patterns. Moreover, we have shown that the visibility difference between the unipolar and the bipolar regime is because of the Klein collimation occurring at a smooth p–n interface in graphene. Our experiment paves the way to more complex engineered ballistic graphene to realize electron lensing, focusing [10] and efficient guiding [8] , [11] . During the review process, we became aware of a related work (‘A ballistic pn junction in suspended graphene with split bottom gates’ by A.L. Grushina, D.-H. Ki and A.F. Morpurgo) that has been published in ref. 32 . Device fabrication Suspended graphene p–n junctions are obtained by combining a mechanical transfer technique with a hydrofluoridric acid-free suspension method developed by Tombros et al . [20] The fabrication starts with the spinning of a polymer stack consisting of a water-soluble polyvinyl alcohol and poly(methyl methacrylate) (PMMA) layer on an oxidized (300 nm) Si wafer, on which alignment markers are predefined. Graphene sheets are then mechanically exfoliated on this stack and located by optical means. Depending on the location of the selected graphene flake, 5/45-nm-thick Ti/Au bottom gate electrodes are tailor-made on a separate oxidized Si wafer by standard e-beam lithography and covered by a 1-μm-thick lift-off resist (LOR), Fig. 3a-1 . Afterwards, the wafer that contains the graphene is immersed in deionized water. Once polyvinyl alcohol is dissolved, the wafer sinks to the bottom, leaving the PMMA-graphene membrane floating on top at the liquid–air interface. Next, this membrane is fished out by a transfer glass, dried and fixed in place of the ultraviolet mask in a modified MJB3 mask aligner. The other wafer, containing the bottom gates and LOR layer, is fixed at the wafer side of the mask aligner. The graphene flake is then carefully aligned to the bottom gates and finally transferred in contact by heating the stack to 120 °C, Fig. 3a-3 . Once transferred, PMMA is dissolved in xylene. Palladium contacts (50 nm in thickness) are then fabricated through PMMA e-beam lithography with xylene as developer and lift-off solvent, Fig. 3a-4 and optical image in Fig. 3b . In the final step, the LOR layer below the graphene is e-beam-exposed and developed in ethyl-lactate to obtain suspended graphene junctions, Fig. 3a-5 . Graphene current annealing After mounting the finished device in a variable temperature 4 He cryostat, we perform current annealing by applying a direct current at 1.5 K. In this procedure, the current is increased until the conductance as a function of a gate voltage V gate shows a pronounced dip around V gate =0 V, reminiscent of a high quality device. This requires current densities that usually reach values up to 350 μA μm −1 . P.R. and R.M. contributed equally to this work. P.R. and R.M. fabricated the devices. Measurements were performed by P.R., R.M., M.W. M.-H.L. performed the conductance simulations and calculations of carrier densities. C.S. guided the experimental part of the work. K.R. guided the theoretical part of the work. All authors worked on the manuscript. How to cite this article: Rickhaus, P. et al . Ballistic interferences in suspended graphene. Nat. Commun. 4:2342 doi: 10.1038/ncomms3342 (2013).